A single-vesicle content mixing assay for SNARE-mediated membrane fusion The in vitro studies of membrane fusion mediated by soluble N -ethylmaleimide-sensitive factor attachment protein receptors (SNAREs) have primarily been conducted by following the mixing of lipids. However, the formation of a fusion pore and its expansion has been difficult to detect directly because of the leakiness of proteoliposomes, vesicle aggregation and rupture that often complicate the interpretation of ensemble fusion experiments. Fusion pore expansion is an essential step for full-collapse fusion and for recycling of fusion mechanisms. Here, we demonstrate a method to detect the inter-vesicular mixing of large cargoes at the single-molecule and -vesicle level. The change in fluorescence resonance energy transfer signal when a DNA hairpin encapsulated in a surface-tethered vesicle encounters a complementary DNA strand from another vesicle indicates content mixing. We found that the yeast SNARE complex alone without any accessory proteins can expand the fusion pore large enough to transmit ~11 kDa cargoes. Membrane fusion underlies a wide variety of cellular activities such as viral infection, fertilization and neurotransmitter release [1] . Synaptic membrane fusion for neurotransmitter release requires a highly conserved protein family termed SNAREs (soluble N -ethylmaleimide-sensitive factor attachment protein receptors) and is regulated by various proteins including synaptotagmins, complexins and SM proteins [2] , [3] . During exocytosis, an incoming vesicle docks to the plasma membrane, apposing membranes are connected by formation of hemifusion stalk, and fusion pores expand to the point at which the vesicle membrane flattens on the plasma membrane surface, leading to the release of complete luminal contents. For an unambiguous dissection of protein-mediated membrane fusion mechanism, in vitro assays were developed on the basis of ensemble lipid mixing of proteoliposomes reconstituted with SNARE proteins. Through these assays, the critical role of SNARE proteins [4] and the importance of different accessory proteins, such as synaptotagmin, complexin and Munc18, as key regulatory factors for the fusion process have been revealed [5] , [6] , [7] . One limitation of the ensemble lipid mixing approach is that it is unable to characterize different stages of fusion, such as docking, hemifusion and full fusion, and has faced some conflicting results from cellular studies [8] . To overcome this limitation, a series of new techniques have been developed for observing lipid mixing of membrane fusion at the single-vesicle level [9] , [10] , [11] , [12] , [13] , [14] . The single-vesicle lipid mixing assay we developed could distinguish between different stages of fusion, such as docking, hemifusion and full fusion through fluorescence resonance energy transfer (FRET) between the donor and acceptor fluorophores incorporated into the separate proteoliposome membranes reconstituted with target membrane SNARE (t-SNARE) or vesicle-SNARE (v-SNARE) proteins [9] . Through our assay, we discovered the stimulatory and inhibitory functions of complexin I [15] and the important role of direct Munc18/SNARE core interaction in promoting lipid mixing [16] . Despite the success with assays based on lipid mixing, they cannot directly detect the content release, which is one of the most rigorous definitions of membrane fusion [17] . Cellular studies showed that content release can proceed through two pathways: kiss-and-run, where a small fusion pore opens transiently on docking of an incoming vesicle, but closes again as the vesicle 'runs' away, and the full-collapse fusion pathway, where the small opening of the pore continues to expand to a large pore [18] , [19] . Unfortunately, both current ensemble and single-vesicle lipid mixing assays are blind to the fusion pore formation and expansion and, therefore, unable to show how the regulatory proteins are involved in this critical step. There is a general assumption that the extent of lipid mixing between vesicles is directly proportional to the extent of content release. However, a recent study on DNA-mediated vesicle fusion showed that highly efficient lipid mixing (up to 80%) of both inner and outer leaflets can occur without mixing of content (less than 2%) [20] . A similar phenomenon was observed with polyethylene glycol (PEG)-mediated membrane fusion [21] . These studies suggest that lipid mixing is necessary for fusion, but lipid mixing alone is an insufficient indicator for full membrane fusion. The original in vitro reconstruction of SNARE-induced membrane fusion used 33 P-labelled oligonucleotides and led to the conclusion that SNARE proteins constitute the minimal machinery for membrane fusion [22] . However, in that study, because the content mixing signal was indirectly measured after vesicles were lysed by the detergent, their result could not clearly separate fusion from vesicle docking and aggregation. Other attempts of using small reporters, such as carboxyfluorescein, for the content mixing studies have mainly failed because of the membrane leakiness after the SNARE protein reconstitution at a physiological protein-to-lipid ratio (>1:500) [21] , unless a very low protein and lipid ratio (<1:1,000) was used [23] , [24] . In this paper, we report the development of a reliable and efficient single-vesicle content mixing assay for SNARE-mediated membrane fusion on the basis of FRET at the single-molecule level [25] . The main advantage of single-molecule experiments here is that fusion events can be clearly distinguished from vesicle aggregation or vesicle rupture. A fluorescently labelled DNA hairpin showed high FRET when it is encapsulated inside a vesicle reconstituted with yeast SNARE proteins. When the vesicle fused with another vesicle containing a complementary DNA strand, FRET decreased to a low level because of the formation of double-stranded DNA. Various control experiments showed that the DNA molecules are inside intact vesicles before and after fusion. The content mixing signal required the functional SNARE complex because removal of Sec9c or its mutations eliminated or reduced the population of vesicles that showed a low FRET signal. Our results established that yeast SNAREs, without any accessory proteins, can induce the formation of fusion pore and can expand the pore to a large enough diameter for ~11 kDa cargoes. SNARE protein-reconstituted vesicles encapsulate DNA probes As SNARE protein reconstitution causes the leakiness of vesicles [21] , a large probe is necessary for a reliable content mixing assay. With inspiration from molecular beacons, we designed a DNA hairpin composed of a 5 bp stem and a polythymidine loop (T 20 ) labelled with a donor (Cy3) and an acceptor (Cy5) fluorophore at either end of the stem ( Supplementary Fig. S1a ). When the loop region of this Cy3/Cy5 dual-labelled DNA probe hybridizes with a second DNA strand having a complementary sequence (A30), the formation of a longer double-strand breaks apart the stem region, which moves the donor and acceptor fluorophores away from one another. As a result of this distance change, the FRET efficiency ( E ) switches from a high to a low value ( Supplementary Fig. S1b and S1c ). Dual-labelled DNA and the complementary polyadenosine (poly-A) strands are encapsulated inside proteoliposomes reconstituted with v-SNARE and t-SNARE, respectively, and the FRET signal is used to monitor the extent of SNARE-mediated content mixing. DNA molecules encapsulated inside vesicles are functional [26] , [27] , [28] , which makes the Cy3/Cy5 dual-labelled DNA probe a viable candidate for a content mixing indicator. Because many earlier attempts suffered from probe leakage, we first tested the stability of our dual-labelled DNA probe inside the vesicle. The details of proteoliposome preparation can be found in the Methods section. Dual-labelled DNA probe-encapsulated vesicles reconstituted with yeast v-SNARE protein (Snc2p) (1:200 protein-to-lipid ratio) were immobilized on the polymer-coated imaging surface. Nonspecific binding of dual-labelled DNA probes outside the vesicle was prevented by polymer, and these DNA molecules were washed away with excess buffer ( Supplementary Fig. S3a ). Single-molecule fluorescence signals from DNA molecules in individual vesicles were collected and plotted as a histogram, showing a distinct high E as expected ( Fig. 1a, left). To verify that these probes were inside the vesicle, deoxyribonuclease I (DNase) was added to the system. The number of molecules showing the high FRET signal before and after treatment did not show a significant difference ( Fig. 1a ) and no shift in E distribution was observed. This shows that DNA probes are inside vesicles and are protected from DNase digestion by the lipid bilayer. In contrast, DNase treatment effectively eliminated DNA probes unprotected by vesicles ( Fig. 1b ). These DNA probes did not leak out of vesicles over the course of 60 min ( Fig. 1c ), and showed a stable high E distribution at 37 °C incubation, as well as in the presence of free poly-A DNA outside the vesicles ( Supplementary Fig. S3b ). These control experiments show that the Cy3/Cy5 dual-labelled DNA probe could be used as a reliable content mixing indicator. 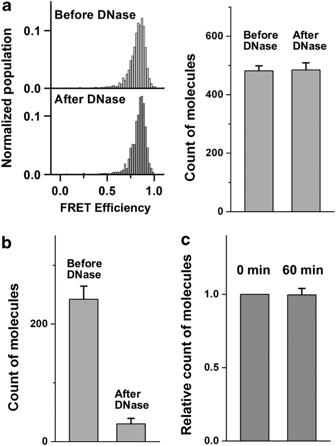Figure 1: Stable encapsulation of DNA probes inside SNARE protein-reconstituted vesicles. (a) Histograms of FRET efficiency,E(left), and average numbers (right) of molecules per imaging area (25×50 μm) before and after DNase treatment of DNA probes encapsulated inside surface-immobilized v-SNARE (protein/lipid=1:200) vesicles. For histograms of FRET efficiency, theyaxis denotes the normalized population, where we divided the distribution by the total number of vesicles measured, and thexaxis denotes the FRET efficiency value. (b) Average count of molecules per imaging area before and after DNase treatment of DNA probes immobilized outside vesicles (corresponding representative images for (a) and (b) are shown inSupplementary Fig. S2). (c) Relative count of molecules per imaging area for surface-immobilized v-vesicle-encapsulating DNA probes after incubating at 37 °C for 60 min. The number of molecules at 0 min was set as 1. Error bars denote the s.e. Figure 1: Stable encapsulation of DNA probes inside SNARE protein-reconstituted vesicles. ( a ) Histograms of FRET efficiency, E (left), and average numbers (right) of molecules per imaging area (25×50 μm) before and after DNase treatment of DNA probes encapsulated inside surface-immobilized v-SNARE (protein/lipid=1:200) vesicles. For histograms of FRET efficiency, the y axis denotes the normalized population, where we divided the distribution by the total number of vesicles measured, and the x axis denotes the FRET efficiency value. ( b ) Average count of molecules per imaging area before and after DNase treatment of DNA probes immobilized outside vesicles (corresponding representative images for ( a ) and ( b ) are shown in Supplementary Fig. S2 ). ( c ) Relative count of molecules per imaging area for surface-immobilized v-vesicle-encapsulating DNA probes after incubating at 37 °C for 60 min. The number of molecules at 0 min was set as 1. Error bars denote the s.e. Full size image Single-vesicle content mixing assay We applied our content mixing assay to the yeast SNAREs (Sso1p, Snc2p and Sec9c) that mediate constitutive fusion of transport vesicles to the plasma membrane [29] . 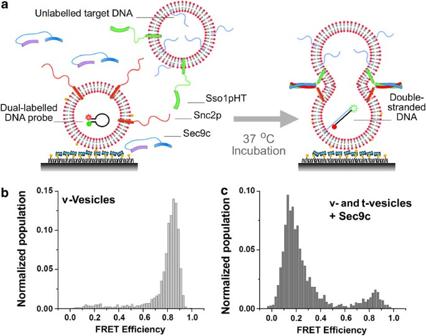Figure 2: Single-molecule content mixing assay for yeast SNARE-mediated fusion. (a) Schematics of the assay. Vesicles reconstituted with Snc2p proteins (v-vesicles) and encapsulating dual-labelled DNA probes are immobilized on the surface of the flow cell. Vesicles reconstituted with Sso1pHT proteins (t-vesicles) and encapsulating poly-A DNA strands are flown in, along with soluble Sec9c proteins, and the sample is incubated at 37 °C. (b)Edistributions of v-vesicles before the reaction, and (c) after incubating for 30 min with t-vesicles and 1 μM Sec9c protein. Figure 2a shows the basic scheme of our assay. v-SNARE vesicles, with Snc2p in the membrane and DNA hairpin encapsulated inside, are immobilized on a polymer-coated quartz surface by means of biotinylated lipids [9] . The t-SNARE vesicles containing Sso1pHT and harbouring multiple poly-A DNAs with a cholesterol modification are added together with soluble Sec9c (1 μM), and the sample is incubated at 37 °C. The average number of dual-labelled DNA probes inside the v-SNARE vesicle quantified from the number of photobleaching steps is ~0.4 ( Supplementary Fig. S4 ). Cholesterol modification increases the incorporation efficiency of poly-A DNA in the t-SNARE vesicle membrane, thus increasing the probability of two vesicles with DNA probes to react ( Supplementary Fig. S5 ). When two vesicles, both ~100 nm in diameter, dock and a large enough fusion pore forms between them, the two DNA molecules should hybridize to switch the E between Cy3 and Cy5 from a high ( Fig. 1a ) to a low value ( Supplementary Fig. S1c ). Figure 2: Single-molecule content mixing assay for yeast SNARE-mediated fusion. ( a ) Schematics of the assay. Vesicles reconstituted with Snc2p proteins (v-vesicles) and encapsulating dual-labelled DNA probes are immobilized on the surface of the flow cell. Vesicles reconstituted with Sso1pHT proteins (t-vesicles) and encapsulating poly-A DNA strands are flown in, along with soluble Sec9c proteins, and the sample is incubated at 37 °C. ( b ) E distributions of v-vesicles before the reaction, and ( c ) after incubating for 30 min with t-vesicles and 1 μM Sec9c protein. Full size image Figure 2b,c shows actual E distributions before and after addition of t-SNARE vesicle/Sec9c to the flow cell and incubation for 30 min at 37 °C. The E distribution measured from thousands of single DNA hairpin probes clearly switched from ~0.8 to ~0.2 ( Fig. 2b,c ). We repeated the same experiment using DNA without the cholesterol link to the target DNA and observed a similar shift in the E distribution, but with a reduced extent of FRET population shift due to a lower DNA encapsulation efficiency ( Supplementary Fig. S5 ). To further ensure that the DNA hybridizations are taking place inside vesicles, the sample was treated with DNase after the fusion reaction. The E distribution remained the same and the average number of fluorescent spots did not decrease, indicating that all observed signals came from DNA probes inside vesicles ( Fig. 3a ). 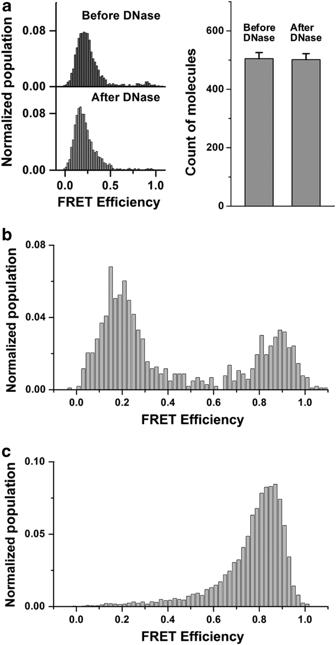Figure 3: Various controls to establish the single-vesicle content mixing assay. (a) DNA annealing takes place inside vesicles.Edistributions (left) and average numbers of molecules per imaging area (25×50 μm) (right) of fusion products before and after DNase treatment. Error bars denote s.e. Corresponding representative images are shown inSupplementary Figure S6. (b)Edistribution of the fusion product with 1 μM Sec9c performed in the bulk solution and subsequently immobilized on the quartz surface for observation. DNase treatment was applied to both v- and t-vesicles to eliminate free DNA molecules before reaction. (c)Edistribution after fusion reaction using non-complementary poly-T DNA inside t-vesicles. Figure 3: Various controls to establish the single-vesicle content mixing assay. ( a ) DNA annealing takes place inside vesicles. E distributions (left) and average numbers of molecules per imaging area (25×50 μm) (right) of fusion products before and after DNase treatment. Error bars denote s.e. Corresponding representative images are shown in Supplementary Figure S6 . ( b ) E distribution of the fusion product with 1 μM Sec9c performed in the bulk solution and subsequently immobilized on the quartz surface for observation. DNase treatment was applied to both v- and t-vesicles to eliminate free DNA molecules before reaction. ( c ) E distribution after fusion reaction using non-complementary poly-T DNA inside t-vesicles. Full size image The DNA hairpin probe used is 30 nucleotides long, with a molecular weight of ~11 kDa, whereas most neurotransmitters are much smaller (~0.1 kDa). A transient opening of fusion pores allows passage of small molecules, but the larger molecular weight probes used here may be difficult to pass. Our assay is most likely to report the content mixing resulting from the stably expanded pore that results from the complete collapse of vesicle membranes. The formation of these stable pores was not caused by the surface immobilization step. We verified this by first performing the fusion reaction in bulk solution, and then immobilizing the product onto the surface. As shown in Figure 3b , the major low FRET peak from DNA hybridization was observed as in the standard experimental scheme. This FRET shift was driven in a DNA sequence-dependent manner—and not by protein or vesicle aggregation—for when we replaced target poly-A DNAs in t-vesicles with non-complementary poly-T DNAs, no FRET switch was observed under the same reaction condition on the surface ( Fig. 3c ). Yeast SNAREs are sufficient to induce content mixing The E shift we observed with our content mixing assay is SNARE dependent. A control experiment without Sec9c showed no change in E , whereas lowering the Sec9c concentration (0.1 μM) reduced the vesicle population with expanded pores ( Fig. 4a ). Interestingly, 0.1 μM Sec9c, corresponding to an ~2:1 Sec9/Sso1 ratio, showed a much lower degree of content mixing than lipid mixing [9] . This seems to suggest that, in some instances, lipid mixing could progress without formation of stable pores across the membrane. A time course study showed a progressive shift from E ~0.8 population to E ~0.2 population over 30 min ( Fig. 4b ). 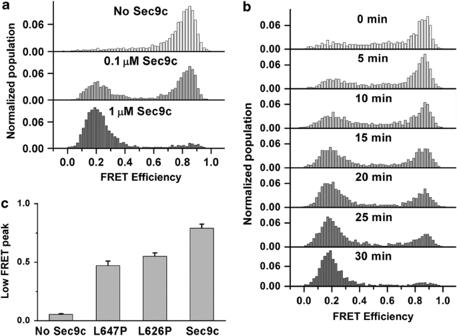Figure 4: Content mixing requires a full SNARE complex with the wild-type Sec9c. (a)Edistributions of fusion products for different Sec9c concentrations. (b)Edistributions of yeast SNARE-mediated fusion with different incubation times ranging from 0 to 30 min with 1 μM Sec9c. (c) Pore expansion efficiency quantified by low FRET peak percentage (E=0–0.4) for wild-type and mutant Sec9c, L626P and L646P. Sec9c (1 μM) and its mutants were used. Error bars denote the s.d. of three independent experiments. A 30 min incubation at 37 °C was applied for all experiments in (a) and (c). Figure 4: Content mixing requires a full SNARE complex with the wild-type Sec9c. ( a ) E distributions of fusion products for different Sec9c concentrations. ( b ) E distributions of yeast SNARE-mediated fusion with different incubation times ranging from 0 to 30 min with 1 μM Sec9c. ( c ) Pore expansion efficiency quantified by low FRET peak percentage ( E =0–0.4) for wild-type and mutant Sec9c, L626P and L646P. Sec9c (1 μM) and its mutants were used. Error bars denote the s.d. of three independent experiments. A 30 min incubation at 37 °C was applied for all experiments in ( a ) and ( c ). Full size image Two helices of Sec9c both contribute to the formation of the four-helix bundle necessary for membrane fusion, but have slightly different roles. The N-terminal helix (SN1) has a more dominant role in the initial docking of the vesicle, whereas the C-terminal helix (SN2) drives the membrane lipid mixing [30] . Helix-breaking proline mutations (L626P, L647P) on the SN2 helix showed a significantly stronger inhibitory effect on the lipid mixing efficiency, compared with the docking efficiency, but their effect on pore formation has been unclear [30] . We tested these mutants using our content mixing assay and found a similar inhibitory effect on the pore formation efficiency ( Fig. 4c ). The proline mutation close to the C-terminal end of the helix (L647P) showed a stronger inhibitory effect than what the L626P mutant did on both lipid and content mixing, supporting the fact that complete engagement of the SN2 helix in the SNARE complex is necessary for completing membrane fusion. A reliable and an efficient content mixing assay based on the FRET switch caused by DNA hybridization has been developed at the single-vesicle level. As the size of our content mixing indicator is much larger than the size of neurontransmitters, fusion pore expansion, the very late step of membrane fusion, is most likely reported through this assay. Yeast SNARE proteins have been known to induce efficient and rapid lipid mixing [31] . Our results further demonstrated that yeast SNARE proteins are necessary and sufficient for expansion of the fusion pore. For the neuronal SNARE on the other hand, although a limited extent of lipid mixing does occur [15] , [21] , [32] , the clear signal of content mixing has not been confirmed yet. Our single-vesicle content mixing assay should be useful in identifying key factors that allow pore expansion in the neuronal SNARE system. Protein preparation Plasmid construction, protein expression and purification for yeast SNAREs were described in detail previously [33] . In brief, Sso1pHT (amino acids 185–290), in which the N-terminal α-helical Habc domain was truncated, and full-length Snc2p (amino acids 1–115) were expressed as the N-terminal glutathione- S -transferase fusion proteins. Sec9c (amino acids 401–651 of Sec9) was expressed as a C-terminal His6-tagged protein. Recombinant proteins were expressed in Escherichia coli Rosetta (DE3) pLysS (Novagen). Glutathione-agarose beads (Sigma) were used to purify Sso1pHT and Snc2p. The protein-bound glutathione- S -transferase beads were washed excessively with washing buffer (phosphate-buffered saline, pH 7.4) containing 0.2% (v/v) Triton X-100. Following the buffer exchange with phosphate-buffered saline (pH 7.4) containing 0.8% (w/v) n -octyl- D -glucopyranoside (OG, Research Product International), the protein of interest was cleaved on a column by thrombin in cleavage buffer (50 mM Tris–HCl, 150 mM NaCl, 0.8% OG, pH 8.0). His6-tagged Sec9c was purified using Ni-NTA agarose beads (Qiagen). The beads were washed with washing buffer (25 mM HEPES, 100 mM KCl with 20 mM immidazole, pH 7.4), and the protein was eluted out by an elution buffer (25 mM HEPES, 100 mM KCl with 150 mM immidazole, pH 7.4). SNARE protein reconstitution The solution of 1-palmitoyl-2-dioleoyl-sn-glycerol-3-phosphatidylcholine, cholesterol and 1,2-dioleoyl-sn-glycero-3-phosphatidylserine (molar ratio of 45:40:15) in chloroform was dried to form a lipid film on the wall of a glass tube. The same procedures and lipid components were applied to prepare another tube of lipid solution, except containing 0.1 mol% biotinylated lipid. The dried lipid film was resuspended with Tris–HCl buffer (10 mM Tris–HCl, 50 mM NaCl, pH 8.0) containing 10 μM target DNAs or 1 μM Cy3–Cy5 dual-labelled DNA probes (Integrated DNA Technologies), separately. After five freeze–thaw cycles, unilamellar vesicles were extruded through polycarbonate filters (100 nm pore size, Avanti Polar Lipids) at least 39 times. Sso1pHT and Snc2p proteins were mixed with vesicles containing target DNAs or vesicles containing dual-labelled DNA probes, separately, at a lipid–protein molar ratio of 200:1. The concentration of OG was kept at 0.8–1% during the reconstitution. After incubation at 4 °C for 20 min, the protein–lipid mixtures were diluted twice to make the concentration of OG below the critical micelle concentration (~0.6%). The mixtures were then dialysed overnight against HEPES buffer (25 mM HEPES/KOH, 100 mM KCl, pH 7.4) at 4 °C. DNase treatment Three units (3 μl) of amplification grade DNase I (Sigma-Aldrich) and 3 μl of 10× reaction buffer (Sigma-Aldrich, 200 mM Tris–HCl, 20 mM MgCl 2 , pH 8.3) were mixed with 24 μl HEPES buffer (25 mM HEPES/KOH, 100 mM KCl, pH 7.4). The treatment was performed at room temperature. Single-molecule content mixing assay For yeast SNARE-mediated fusion, a quartz slide was first coated with PEG molecules (99:1 (mol/mol) mPEG-SVA/biotin-PEG-SVA (Laysan Bio) to eliminate nonspecific binding of vesicles and DNAs [34] . The slide was then assembled into a flow chamber and coated with neutravidin by flowing in 0.2 mg ml −1 solution. Through the specific interaction between biotin and neutravidin, the v-SNARE (Snc2p) vesicles with dual-labelled DNA hairpin probes encapsulated inside were immobilized on the PEG-coated surface by an incubation at vesicle concentration of 100–160 pM for 15 min. After washing out the free v-SNARE vesicles in the chamber, the t-SNARE (Sso1pHT) vesicles containing unlabelled single-strand target DNAs were diluted to a final vesicle concentration of 200 pM with 1 μM Sec9c, and injected into the flow cell for reaction at 37±2 °C in buffer (25 mM HEPES, 100 mM KCl, pH 7.4) for 30 min. After washing out free t-SNARE vesicles and Sec9c proteins, FRET measurements using a total internal reflection (TIR) fluorescence microscope were taken at the thirty-fifth minute by injection of t-SNARE vesicles with an oxygen scavenger system (0.1 mg ml −1 glucose oxidase, 0.02 mg ml −1 catalase and 0.4% (wt/wt) β- D -glucose) and Trolox to eliminate single-molecule blinking events [35] . TIR fluorescence microscope imaging Details of the wide-field TIR fluorescence microscope have been reported [34] . Briefly, the excitation beam was focused into a pellin broca prism (CVI Laser), which was placed on top of a quartz slide with a thin layer of immersion oil in between to match the index of refraction. Cy3 (donor) and Cy5 (acceptor) dyes were excited through the alternating laser excitation system (532 and 633 nm) through TIR. The fluorescence signals from Cy3 and Cy5 that were collected by a water immersion objective lens (60×, 1.2 N.A. Olympus) went through a notch filter to block out excitation beams. The emission signals of Cy5 dyes were separated by a 630 nm dichroic mirror (630DCXR, Chroma Technology) and detected by the electron-multiplying charge-coupled device camera (iXon DV 887-BI, Andor Technology) with a time resolution of 100 ms. Each movie was taken for 10 frames (1 s) with 532 nm excitation, followed by five frames (0.5 s) with 633 nm excitation. The fluorescence signal, recorded in real time by using software written in Visual C++ (Microsoft), was amplified before camera readout, which produced an arbitrary unit for the recorded fluorescence intensity. Single-molecule data analysis Single-molecule data analysis was carried out by programs written in Matlab (MathWorks) and Origin (OriginLab). The FRET efficiency, E , was approximated by the intensity of the acceptor channel divided by the total intensity, which is the sum of donor and acceptor channel intensities. To exclude donor-only molecules, single-vesicle spots were identified by red laser excitation through software written in Visual C++ (Microsoft). How to cite this article: Diao, J. et al . A single-vesicle content mixing assay for SNARE-mediated membrane fusion. Nat. Commun. 1:54 doi: 10.1038/ncomms1054 (2010).